The subcortical maternal complex controls symmetric division of mouse zygotes by regulating F-actin dynamics Maternal effect genes play critical roles in early embryogenesis of model organisms where they have been intensively investigated. However, their molecular function in mammals remains largely unknown. Recently, we identified a subcortical maternal complex (SCMC) that contains four proteins encoded by maternal effect genes ( Mater , Filia , Floped and Tle6 ). Here we report that TLE6, similar to FLOPED and MATER, stabilizes the SCMC and is necessary for cleavage beyond the two-cell stage of development. We document that the SCMC is required for formation of the cytoplasmic F-actin meshwork that controls the central position of the spindle and ensures symmetric division of mouse zygotes. We further demonstrate that the SCMC controls formation of the actin cytoskeleton specifically via Cofilin, a key regulator of F-actin assembly. Our results provide molecular insight into the physiological function of TLE6, its interaction with the SCMC and their roles in the symmetric division of the zygote in early mouse development. During cleavage-stage mouse development, cells divide without a dramatic increase in the overall size of embryos that remain constrained by the extracellular zona pellucida. The actin cytoskeleton (F-actin) plays a fundamental role in dividing cells [1] and pharmacological intervention that disrupts the integrity of the actin cytoskeleton adversely, affects mouse fertilization and early cell division [2] , [3] , [4] . It has recently been reported that the cytoplasmic F-actin meshwork is required to maintain the mitotic spindle in the centre of the zygotes to ensure symmetric division of early mouse embryos [5] . Although well-documented in somatic cells and other model organisms, the regulators of the actin cytoskeleton in mammalian zygotes, remain largely unknown. Given the absence of transcription, it is anticipated that oocyte-stored actin regulators, encoded by maternal genes, will play critical roles in controlling formation of the actin cytoskeleton in cleavage-stage mouse development. Maternal effect genes are essential for early embryonic development prior to zygote gene activation [6] . The pioneering research conducted in Drosophila as early as 1980 (ref. 7 ), and then widely extended to other model systems, well document their essential roles in early embryonic development [8] , [9] , [10] , [11] . However, it was not until 2000 that the first two maternal effect genes were serendipitously discovered in mouse [12] , [13] . Although maternal effect genes are hypothesized to control turnover of maternal RNA and protein, activation of the embryonic genome, cell proliferation and cleavage-stage embryonic development, the molecular mechanism of these genes has not been well documented in mammals. We recently identified a subcortical maternal complex (SCMC) uniquely expressed in mammalian oocytes and early embryos [14] . The SCMC includes at least four proteins: FLOPED (official gene symbol, Ooep ), MATER (official gene symbol, Nlrp5 ) and transducin-like enhancer of split 6 (TLE6, Tle6 ) that bind to each other, as well as FILIA (official gene symbol, Khdc3 ) that binds only to MATER [14] . The genes encoding all four proteins are expressed during oogenesis and their proteins accumulate in growing oocytes and persist in cleavage-stage embryos [14] , [15] , [16] , [17] . Because it is excluded from regions of cell–cell contact, the SCMC becomes polarized to the subcortex underlying the free surface of external cells in cleavage-stage embryos [16] . Null mutations of the single copy genes encoding Mater and/or Floped result in cleavage-stage embryonic arrest and female sterility [12] , [14] . The absence of Filia has a more subtle phenotype with delayed pre-implantation development and decreased fecundity [18] . The presence of MATER and/or FLOPED (but not FILIA) is required for the formation of the SCMC [14] , [18] . Less is known about the role of TLE6 in early mouse development. TLE6 belongs to the Groucho/TLE transcriptional co-repressor family that was first identified as a target of E2A-hepatic leukaemia factor, and is widely expressed in mouse embryos and adult tissues [19] . In neural progenitors, TLE6 antagonizes TLE1 repression by competing with TLE1 binding to brain factor 1 (BF-1) [20] . Tle6 is highly expressed in the newborn ovary and its protein combines with MATER, FLOPED and FILIA to form the SCMC [14] . Although TLE family proteins were documented as the transcriptional co-repressors in signalling pathways (Notch, Wnt, Hedgehog and Dpp/BMP) [21] , defining the physiological functions of these proteins has been difficult because multiple family members are broadly co-expressed in a variety of tissues, which complicates interpretation of genetic loss-of-function studies [22] . In the present investigation, we report that Tle6 is a maternal effect gene required for cleavage-stage embryogenesis. Tle6 Null mice are sterile, and the protein product of Tle6 is required for formation of SCMC in mouse oocytes and early embryos. Most importantly, we document a role for the SCMC as an oocyte–embryo-specific protein complex that controls symmetric division of mouse zygotes by regulating the actin cytoskeleton through Cofilin. Localization of the SCMC in mouse oocytes and early embryos Individual proteins of the SCMC were observed in the subcortex of eggs and early embryos after whole mount staining with specific antibodies [14] , [15] , [16] , [17] , [23] , [24] . However, two components (MATER and FLOPED) were additionally detected throughout the cytoplasm of eggs and embryos when the staining was performed after fixation with paraformaldehyde and embedding in paraffin [23] , [24] . To investigate the potential problem of antibody accessibility, which was proposed to account for this discrepancy [23] , [24] , we examined the localization of TLE6, FLOPED and MATER with paraffin sections of mouse early embryos. To avoid potential artifacts from embedding in agarose, we fixed mouse early embryos in the oviduct and prepared paraffin sections for staining. Consistent with the results from previous whole mount studies [14] , [15] , [16] , [17] , [23] , [24] , TLE6, FLOPED and MATER were primarily present in the subcortex of mouse zygotes in paraffin sections ( Fig. 1a–c ). In particular, TLE6 was primarily located in the subcortical domain of two-cell and morular stage embryos that were fixed in the oviduct, embedded in paraffin and sectioned ( Supplementary Fig. 1a ). The subcortical localization of TLE6 was further confirmed by the injection of mouse zygotes with messenger RNA (mRNA) encoding enhanced green fluorescent protein (eGFP)-tagged TLE6 ( Supplementary Fig. 1b and Supplementary Movie 1 ). 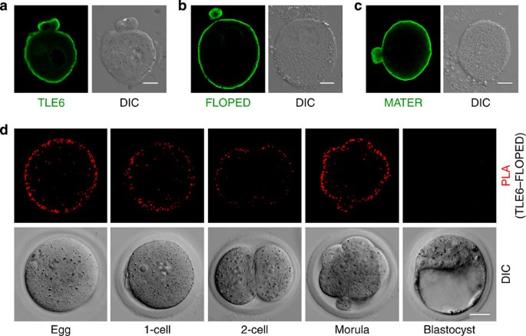Figure 1: Expression of the SCMC in mouse eggs and early embryos. (a) Mouse zygotes were fixed in the oviduct, embedded in paraffin and sectioned (4 μm). The sections were stained with rabbit anti-TLE6 and imaged with confocal microscopy. Scale bar, 20 μm. (b) Same asa, but with rabbit anti-FLOPED antibodies. (c) Same asa, but with rabbit anti-MATER antibodies. (d) The location and proximity of FLOPED and TLE6 in eggs and zygotes from normal females were determined with a proximity ligation assay (PLA) using rabbit anti-FLOPED and anti-TLE6 antibodies. After staining, the eggs/embryos were imaged by confocal and differential interference contrast (DIC) microscopy. Scale bar, 20 μm. Figure 1: Expression of the SCMC in mouse eggs and early embryos. ( a ) Mouse zygotes were fixed in the oviduct, embedded in paraffin and sectioned (4 μm). The sections were stained with rabbit anti-TLE6 and imaged with confocal microscopy. Scale bar, 20 μm. ( b ) Same as a , but with rabbit anti-FLOPED antibodies. ( c ) Same as a , but with rabbit anti-MATER antibodies. ( d ) The location and proximity of FLOPED and TLE6 in eggs and zygotes from normal females were determined with a proximity ligation assay (PLA) using rabbit anti-FLOPED and anti-TLE6 antibodies. After staining, the eggs/embryos were imaged by confocal and differential interference contrast (DIC) microscopy. Scale bar, 20 μm. Full size image Proximity ligation assays (PLA) provide highly specific and sensitive in situ detection of protein interactions within a complex [25] . Therefore, to further investigate the SCMC in mouse oocytes and early embryos, we developed a PLA by using probe-conjugated rabbit anti-TLE6 and -FLOPED antibodies. The SCMC was primarily detected in the subcortex of mouse eggs and early embryos and had largely disappeared in early blastocysts ( Fig. 1d and Supplementary Fig. 1c ). Surprisingly, although the abundance of TLE6 and FLOPED detected by immunoblot and immunofluorescence was similar in eggs and early embryos [14] , [15] , [16] , [17] , the SCMC detected by the PLA was more abundant and concentrated in eggs, zygotes and morulae than in two-cell embryos ( Fig. 1d and Supplementary Fig. 1c ). The dynamic changes of the SCMC in mouse oocytes and early embryos raised the possibility that the SCMC function may vary depending on the embryonic stage. These results substantiate the primary localization of the SCMC in the subcortex of mouse eggs and early embryos. Establishing and characterizing Tle6 Null mice To investigate the physiological function of TLE6, a mouse strain lacking this protein was generated ( Supplementary Fig. 1d–f ). F 1 Tle6 +/− female and male mice produced 24 litters with a total of 166 offspring, the genotypes of which (46 Tle6 +/+ , 28%; 80 Tle6 +/− , 48%; 40 Tle6 −/− , 24%) were consistent with the expected Mendelian frequency (1:2:1). Tle6 +/− and Tle6 −/− mice grew normally to adulthood. Unless otherwise stated, Tle6 +/− ( Mater +/− , Floped +/− ) and Tle6 −/− ( Mater −/− , Floped −/− ) will be referred to as control and Tle6 Null ( Mater Null , Floped Null ), respectively. SCMC null mice refer collectively to Tle6 Null , Mater Null and Floped Null females. Tle6 transcripts were absent in Tle6 Null ovaries ( Fig. 2a ) and TLE6 protein was not detected in Tle6 Null eggs ( Fig. 2b,c ). Although Tle6 is expressed early in mouse ovaries [14] , Tle6 Null females had normal ovarian histology in which all stage follicles were present ( Fig. 2d ). After administration of gonadotrophins to stimulate ovulation, the number and morphology of eggs recovered from Tle6 Null females were comparable to those obtained from control female mice ( Fig. 2e and Supplementary Fig. 1g ). However, after mating for 3 months with normal males proven fertility, Tle6 Null female mice produced no offspring ( Table 1 ). Thus, while not essential for oogenesis and ovulation, TLE6 is required for the fertility of female mice. 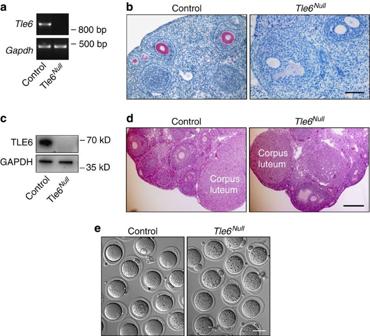Figure 2: Characterization ofTle6mutant mice. (a)Tle6transcripts were detected in control (+/−), but notTle6Nullovaries by semi-quantitative RT–PCR usingGapdhas a control for integrity of sample RNA. (b) TLE6 protein was detected in control, but not inTle6Nullovaries by immunohistochemistry using rabbit anti-TLE6 antibodies. Scale bar, 100 μm. (c) TLE6 protein was detected in control (+/−), but notTle6Null, egg lysates by immunoblot using antibodies to TLE6 and GAPDH (loading control). (d) Ovarian histology of control andTle6Nullovaries after staining with periodic acid-Schiff’s (PAS) reagent. Scale bar, 200 μm. (e) DIC images of ovulated eggs from control andTle6Null. Scale bar, 20 μm. Figure 2: Characterization of Tle6 mutant mice. ( a ) Tle6 transcripts were detected in control (+/−), but not Tle6 Null ovaries by semi-quantitative RT–PCR using Gapdh as a control for integrity of sample RNA. ( b ) TLE6 protein was detected in control, but not in Tle6 Null ovaries by immunohistochemistry using rabbit anti-TLE6 antibodies. Scale bar, 100 μm. ( c ) TLE6 protein was detected in control (+/−), but not Tle6 Null , egg lysates by immunoblot using antibodies to TLE6 and GAPDH (loading control). ( d ) Ovarian histology of control and Tle6 Null ovaries after staining with periodic acid-Schiff’s (PAS) reagent. Scale bar, 200 μm. ( e ) DIC images of ovulated eggs from control and Tle6 Null . Scale bar, 20 μm. Full size image Table 1 Fertility of Tle6 Null female. Full size table The function of TLE6 in mouse early embryogenesis Given its maternal expression, we investigated the potential role of TLE6 in mouse pre-implantation development. Tle6 Null females were mated with normal males, and the embryos were recovered at E0.5 (embryonic day 0.5), E1.5, E2.5 and E3.5. The number of one-cell embryos recovered from Tle6 Null female mice at E0.5 was comparable to the controls ( Fig. 3a,b ). Compared with the control, the progression from one- to two-cell embryos was delayed by 4–6 h ( Supplementary Fig. 1h ). At E2.5 and E3.5, when embryos from the control developed into morulae and blastocysts, respectively, the embryos from Tle6 Null female mice developed into fragmented cytoplasmic blebs ( Fig. 3a,b ). These data demonstrate that TLE6 is essential for mouse pre-implantation embryonic development. 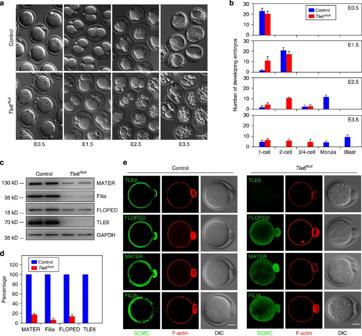Figure 3: The effect of TLE6 on early mouse embryogenesis. (a) After hormonal stimulation andin vivomating with normal males, embryos were flushed from the oviduct of control andTle6Nullfemale mice at E0.5, E1.5, E2.5 and E3.5 and imaged by DIC. Scale bar, 50 μm. (b) The number (mean±s.e.m.) of embryos flushed from the oviducts of more than five controls andTle6Nullfemale mice at E0.5, E1.5, E2.5 and E3.5. after hormonal stimulation and mating with normal male mice. (c) Immunoblot of egg (20) lysates from control andTle6Nullfemale mice probed with antibodies to MATER, Filia, FLOPED, TLE6 and GAPDH. (d) The abundance (mean±s.e.m.) of the SCMC components in control andTle6Nulleggs (20) was determined by immunoblot using four independent samples from each group and setting protein abundance at 100% for control eggs. (e) Localization of TLE6, MATER, FLOPED and FILIA in ovulated eggs from control andTle6Nullfemales was determined by confocal microscopy and DIC. Phalloidin labelled with Alex Fluor 546 was used to detect F-actin. Scale bar, 20 μm. Figure 3: The effect of TLE6 on early mouse embryogenesis. ( a ) After hormonal stimulation and in vivo mating with normal males, embryos were flushed from the oviduct of control and Tle6 Null female mice at E0.5, E1.5, E2.5 and E3.5 and imaged by DIC. Scale bar, 50 μm. ( b ) The number (mean±s.e.m.) of embryos flushed from the oviducts of more than five controls and Tle6 Null female mice at E0.5, E1.5, E2.5 and E3.5. after hormonal stimulation and mating with normal male mice. ( c ) Immunoblot of egg (20) lysates from control and Tle6 Null female mice probed with antibodies to MATER, Filia, FLOPED, TLE6 and GAPDH. ( d ) The abundance (mean±s.e.m.) of the SCMC components in control and Tle6 Null eggs (20) was determined by immunoblot using four independent samples from each group and setting protein abundance at 100% for control eggs. ( e ) Localization of TLE6, MATER, FLOPED and FILIA in ovulated eggs from control and Tle6 Null females was determined by confocal microscopy and DIC. Phalloidin labelled with Alex Fluor 546 was used to detect F-actin. Scale bar, 20 μm. Full size image TLE6 participates in the SCMC, and the phenotype of Tle6 Null female was similar to those of Floped Null and Mater Null females [12] , [14] . Therefore, eggs from control and Tle6 Null females were examined by immunoblot and immunostaining with specific antibodies to individual components of the SCMC. Compared with the protein levels in the control, MATER, Filia and FLOPED were significantly decreased in the eggs from Tle6 Null mice ( Fig. 3c–e ). In addition, individual components of the SCMC were diffusely present in Tle6 Null eggs, except for TLE6 itself which was absent, while the same proteins were primarily present in the subcortex of control eggs ( Fig. 3e ). Because we did not detect significant difference in the mRNA of Mater , Floped and Filia between control and Tle6 Null ovaries, we conclude that TLE6 is required for the stability of the SCMC. The SCMC controls the spindle position in mouse zygotes Most embryos recovered from control female mice at E1.5 formed two, equal-size blastomeres. In striking contrast, over 90% of two-cell embryos from Tle6 Null female mice had unequal-sized blastomeres ( Figs 3a and 4a ). A similar phenotype was observed in embryos from Floped Null and Mater Null females [14] ( Fig. 4a ), raising the possibility that TLE6, and by extension the SCMC, might be required for the symmetric division of mouse zygote. 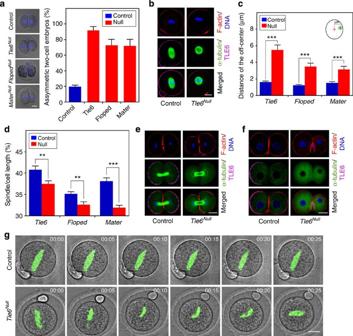Figure 4: Disrupted SCMC affects zygote cleavage and spindle function. (a) Embryos were flushed from the oviduct of five SCMC mutant or control females at E1.5 and stained with Hoechest 33342. Size of each blastomere was calculated by the area of central optical section. The embryo was regarded as asymmetric when the ratio of blastomere sizes in one embryo varied by >10%. Left panel showed DIC images with DNA staining from control and SCMCNullzygotes. Right panel showed percentage (mean±s.e.m.) of asymmetric divisions by using four to five independent samples (Tle6Null, 4;FlopedNull, 5;MaterNull, 4). (b) Zygotes were isolated fromTle6+/−(control) andTle6Nullfemales 28–29 h and 32–33 h after hCG, respectively, cultured for 2–3 h to metaphase and stained with FITC-labelled α-tubulin antibody phalloidin labelled with Alexa Fluor 546 (F-actin), Hoechest 33342 and TLE6 antibody. Scale bar, 20 μm. (c) Zygotes from control andTle6Nullfemales were stained as inb. Spindle position was determined by the distance (d, mean±s.e.m.) from the centre (red cross) of zygotes (circle) to the central chromosome (blue line) in their spindle (small oval). The zygote number for each group:Tle6+/−(n=32),Tle6Null(n=35);Floped+/−(n=50),FlopedNull(n, 38);Mater+/−(n=51),MaterNull(n=42). ***P<0.001 indicates statistically significant differences using Student’st-test. (d) Zygotes from control and null females were treated as inbto determine relative length (mean±s.e.m.) of spindle at metaphase. Spindle size in control (Tle6+/−,n=37;Floped+/−,n=62;Mater+/−,n=44) and null zygotes (Tle6Null,n=35;FlopedNull,n=37;MaterNull,n=41) are reported as ratio (%) of the spindle to cell length. Student’st-test was used to test the statistical differences between controls and SCMCNullzygotes. **P<0.01; ***P<0.001. (e) Zygotes from control andTle6Nullfemales were cultured to telophase and stained as inb. Scale bar, 20 μm. (f) Two-cell embryos were stained as inb. Scale bar, 20 μm. (g) Zygotes from control andTle6Nullwere microinjected with β5-tubulin mRNA, cultured for 4–8 h and imaged with the UltraVIEW VoX system to detect spindle movement. Images are representative frames from control (Supplementary Movie 2) andTle6Null(Supplementary Movie 3) mouse zygotes. Scale bar, 20 μm. Figure 4: Disrupted SCMC affects zygote cleavage and spindle function. ( a ) Embryos were flushed from the oviduct of five SCMC mutant or control females at E1.5 and stained with Hoechest 33342. Size of each blastomere was calculated by the area of central optical section. The embryo was regarded as asymmetric when the ratio of blastomere sizes in one embryo varied by >10%. Left panel showed DIC images with DNA staining from control and SCMC Null zygotes. Right panel showed percentage (mean±s.e.m.) of asymmetric divisions by using four to five independent samples ( Tle6 Null , 4; Floped Null , 5; Mater Null , 4). ( b ) Zygotes were isolated from Tle6 +/− (control) and Tle6 Null females 28–29 h and 32–33 h after hCG, respectively, cultured for 2–3 h to metaphase and stained with FITC-labelled α-tubulin antibody phalloidin labelled with Alexa Fluor 546 (F-actin), Hoechest 33342 and TLE6 antibody. Scale bar, 20 μm. ( c ) Zygotes from control and Tle6 Null females were stained as in b . Spindle position was determined by the distance ( d , mean±s.e.m.) from the centre (red cross) of zygotes (circle) to the central chromosome (blue line) in their spindle (small oval). The zygote number for each group: Tle6 +/− ( n =32), Tle6 Null ( n =35); Floped +/− ( n =50), Floped Null (n, 38); Mater +/− ( n =51), Mater Null ( n =42). *** P <0.001 indicates statistically significant differences using Student’s t -test. ( d ) Zygotes from control and null females were treated as in b to determine relative length (mean±s.e.m.) of spindle at metaphase. Spindle size in control (Tle6 +/− , n =37; Floped +/− , n =62; Mater +/− , n =44) and null zygotes ( Tle6 Null , n =35; Floped Null , n =37; Mater Null , n =41) are reported as ratio (%) of the spindle to cell length. Student’s t -test was used to test the statistical differences between controls and SCMC Null zygotes. ** P <0.01; *** P <0.001. ( e ) Zygotes from control and Tle6 Null females were cultured to telophase and stained as in b . Scale bar, 20 μm. ( f ) Two-cell embryos were stained as in b . Scale bar, 20 μm. ( g ) Zygotes from control and Tle6 Null were microinjected with β5-tubulin mRNA, cultured for 4–8 h and imaged with the UltraVIEW VoX system to detect spindle movement. Images are representative frames from control ( Supplementary Movie 2 ) and Tle6 Null ( Supplementary Movie 3 ) mouse zygotes. Scale bar, 20 μm. Full size image Therefore, spindles in the zygotes from control and SCMC mutant females were examined with FITC-labelled mouse anti-α-tubulin antibody. Compared with controls, the mitotic spindles from SCMC mutant females were dysmorphic, smaller and significantly displaced from the cell centre ( Fig. 4b,c ; Supplementary Fig. 2a,b ). Because the spindle sizes were observed to be significantly different among mouse lines, we compared spindle size using the embryos from heterozygous female of each line as controls. The spindle sizes in mutant zygotes were significantly smaller than those in controls ( Fig. 4d ). Consistent with acentric spindles, the SCMC mutant embryos divided asymmetrically at telophase stage ( Fig. 4e ; Supplementary Fig. 2a,b ), resulting in embryos with unequal-sized blastomeres at the two-cell stage ( Fig. 4f ; Supplementary Fig. 2a,b ). Thus, the percentage of unequally divided embryos was significantly higher in the SCMC mutant mice compared with the control when assayed in vivo or in vitro ( Fig. 4a and Supplementary Fig. 2c,d ). To further investigate spindle formation, one-cell embryos from control or Tle6 Null females were injected with mRNA encoding β5-tubulin–GFP [26] and cultured for live imaging. 34% (84/251) of normal and 30% (150/502) of Tle6 Null zygotes survived microinjection and of these, 42% (34/84) of normal and 27% (40/149) of the Tle6 Null zygotes progressed through nuclear envelope breakdown. In total, 82% (28/34) of normal and 63% (17/27) of the Tle6 Null zygotes were successfully labelled for live imaging of spindle morphology. Typical spindle morphology was observed in all of the normal zygotes ( n =28) and in none of the Tle6 Null zygotes ( n =17; Fig. 4g , Supplementary Movies 2 and 3 ). Compared with controls, spindle orientation was significantly altered ( Fig. 4g ; 10/17, 58%), which suggests that spindle movement is a major cause for acentric spindle localization in Tle6 Null zygotes ( Fig. 4b,c ). Collectively, the above analyses document that the SCMC is required for spindle formation and its position in mouse zygotes. The SCMC regulates cytoskeleton dynamics in mouse zygotes The cytoplasmic F-actin meshwork controls the central spindle position in mouse zygotes [5] . To explore the potential role of the SCMC in centring the spindle, mitotic zygotes from normal and Tle6 Null female mice were stained with fluorescence-labelled phalloidin. Consistent with this earlier report, F-actin was primarily present in the subcortex and formed a meshwork in normal mitotic zygotes ( Fig. 5a ). However, the cytoplasmic F-actin didn't form the fine meshwork in zygotes from Tle6 Null female mice ( Fig. 5b ; Supplementary Fig. 3a ). The cytoplasmic F-actin meshwork was further investigated by live imaging of F-actin with UtrCH–eGFP [27] , which confirmed the absence of F-actin meshwork in Tle6 Null embryos ( Fig. 5c ; Supplementary Movies 4 and 5 ). A similar phenotype was observed in the cytoplasm of zygotes from Mater Null and Floped Null females ( Supplementary Fig. 3b,c ). Together, these data suggest that the SCMC controls spindle position through the cytoplasmic F-actin meshwork in mouse zygotes. 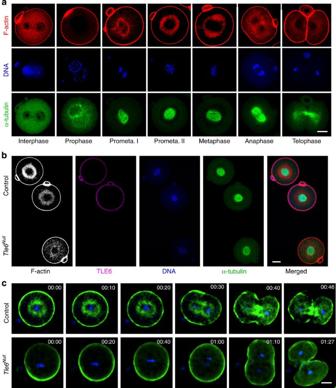Figure 5: Disruption of the SCMC affects the cytoplasmic F-actin meshwork in mouse zygotes. (a) Zygotes were recovered from normal females 28–29 h after hCG, and cultured to different mitotic stages. After fixation and staining with FITC-labelled mouse anti-α-tubulin, phalloidin labelled with Alexa Fluor 546 (F-actin) and Hoechst 33342 (DNA), the embryos were imaged by confocal microscopy. Scale bar, 20 μm. (b) Zygotes were isolated from control as inaandTle6Nullfemales 32–33 h after hCG, and cultured to mitotic stages. After fixation, the embryos of control andTle6Nullembryos were stained as ina. A grey Indicator in colour LUTs was used to show the cytoplasmic F-actin. Scale bar, 20 μm. (c) Zygotes from normal mice andTle6Nullmice were injected with UtrCH–eGFP mRNA and imaged with the UltraVIEW VoX confocal imaging system. Representative images were from control (Supplementary Movie 4) andTle6Null(Supplementary Movie 5) zygotes. Hoechest 33342 was used to stain DNA. Scale bar, 20 μm. Figure 5: Disruption of the SCMC affects the cytoplasmic F-actin meshwork in mouse zygotes. ( a ) Zygotes were recovered from normal females 28–29 h after hCG, and cultured to different mitotic stages. After fixation and staining with FITC-labelled mouse anti-α-tubulin, phalloidin labelled with Alexa Fluor 546 (F-actin) and Hoechst 33342 (DNA), the embryos were imaged by confocal microscopy. Scale bar, 20 μm. ( b ) Zygotes were isolated from control as in a and Tle6 Null females 32–33 h after hCG, and cultured to mitotic stages. After fixation, the embryos of control and Tle6 Null embryos were stained as in a . A grey Indicator in colour LUTs was used to show the cytoplasmic F-actin. Scale bar, 20 μm. ( c ) Zygotes from normal mice and Tle6 Null mice were injected with UtrCH–eGFP mRNA and imaged with the UltraVIEW VoX confocal imaging system. Representative images were from control ( Supplementary Movie 4 ) and Tle6 Null ( Supplementary Movie 5 ) zygotes. Hoechest 33342 was used to stain DNA. Scale bar, 20 μm. Full size image The SCMC co-localizes with F-actin in the subcortex of mouse eggs and early embryos, and the defect of F-actin in SCMC null zygotes raised the possibility that the SCMC directly regulates subcortical F-actin. To address this question, the oocytes and zygotes (pronuclear stages 5) from control (heterozygote) and SCMC mutant ( Tle6 Null , Mater Null , Floped Null ) female mice were paired and F-actin was stained with fluorescence-labelled phalloidin and mouse anti-pan-actin antibody. The immunofluorescent intensity of subcortical F-actin in eggs from Tle6 Null female was similar to that in controls ( Supplementary Fig. 4a,b ). The subcortical F-actin was further investigated by injecting oocytes with the mRNA encoding UtrCH–eGFP, which was recently used to detect the thickness of subcortical F-actin in mouse oocytes [28] . Compared with controls, the thickness of subcortical F-actin was no different in Tle6 Null oocytes at different stages ( Supplementary Fig. 4c,d ). However, the immunofluorescent intensity of subcortical F-actin in zygotes was significantly decreased in SCMC mutant female mice compared with controls ( Fig. 6a,b and Supplementary Fig. 5a,b ). The thickness of subcortical F-actin detected by UtrCH–eGFP was also significantly decreased in the zygotes from Tle6 Null females ( Fig. 6c,d ). In a complementary manner, cytoplasmic G-actin detected with Alex488-DNase I was significantly increased in zygotes from SCMC mutant females, and thickened F-actin bundles were observed in their cytoplasm ( Fig. 6e and Supplementary Fig. 5c,d ). These results suggest that the SCMC regulates the actin dynamics by controlling subcortical F-actin in mouse zygotes. 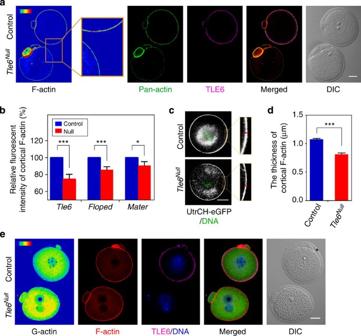Figure 6: The SCMC is required for the assembly of subcortical F-actin in mouse zygotes. (a) Mouse zygotes at similar developmental stages (interphase) were recovered from control andTle6Nullfemales 28–29 h and 32–33 h after hCG, respectively. After fixation, the embryos were mixed and stained with mouse anti-pan-actin, rabbit anti-TLE6 antibodies and phalloidin labelled with Alexa Fluor 546. TLE6 staining was used to distinguish zygotes from control andTle6Nullfemales. F-actin was labelled with phalloidin (red) and used a Rainbow Indicator in colour LUTs to depict the intensity of fluorescence, which was shown in the inserted picture. Scale bar, 20 μm. (b) Paired zygotes from control (heterozygote) and null (Tle6Null,FlopedNullorMaterNull) females were stained with fluorescently labelled phalloidin and specific antibodies to TLE6, FLOPED and MATER, which were used to separate the zygotes from control or null females. The immunofluorescence intensity of subcortical F-actin was analyzed with ZEN lite 2011. The intensity of subcortical F-actin in controls was set as 100%. The number of paired embryos was 47 forTle6, 22 forFlopedand 46 forMater. Error bars represents s.e.m. *P<0.05; ***P<0.001 indicates statistically significant differences using Student’st-test. (c) Zygotes from control andTle6Nullfemales were microinjected with UtrCH–eGFP mRNA, cultured for 4–5 h and imaged with UltraVIEW VoX confocal system at the pronuclear stage. Enlarged images (X3) of the control andTle6Nullzygotes indicated the thickness of cortical F-actin. The red bar showed the thickness of cortical F-actin. Scale bar, 20 μm. (d) Bar graph (mean±s.e.m.) of cortical F-actin thickness at mitotic zygotes from control andTle6Nullfemales. Embryo number was 25 (control) or 20 (Tle6Null). ***P<0.001 indicates statistically significant differences using Student’st-test. (e) Mouse zygotes from control andTle6Nullfemales were recovered as inaand stained with DNase I labelled with Alexa Fluor 488 (G-actin, green), phalloidin labelled with Alexa Fluor 546 (F-actin, red) and rabbit anti-TLE6 antibody (TLE6, magenta). G-actin was used as a Rainbow Indicator to depict the intensity of fluorescence. Scale bar, 20 μm. Figure 6: The SCMC is required for the assembly of subcortical F-actin in mouse zygotes. ( a ) Mouse zygotes at similar developmental stages (interphase) were recovered from control and Tle6 Null females 28–29 h and 32–33 h after hCG, respectively. After fixation, the embryos were mixed and stained with mouse anti-pan-actin, rabbit anti-TLE6 antibodies and phalloidin labelled with Alexa Fluor 546. TLE6 staining was used to distinguish zygotes from control and Tle6 Null females. F-actin was labelled with phalloidin (red) and used a Rainbow Indicator in colour LUTs to depict the intensity of fluorescence, which was shown in the inserted picture. Scale bar, 20 μm. ( b ) Paired zygotes from control (heterozygote) and null ( Tle6 Null , Floped Null or Mater Null ) females were stained with fluorescently labelled phalloidin and specific antibodies to TLE6, FLOPED and MATER, which were used to separate the zygotes from control or null females. The immunofluorescence intensity of subcortical F-actin was analyzed with ZEN lite 2011. The intensity of subcortical F-actin in controls was set as 100%. The number of paired embryos was 47 for Tle6 , 22 for Floped and 46 for Mater . Error bars represents s.e.m. * P <0.05; *** P <0.001 indicates statistically significant differences using Student’s t -test. ( c ) Zygotes from control and Tle6 Null females were microinjected with UtrCH–eGFP mRNA, cultured for 4–5 h and imaged with UltraVIEW VoX confocal system at the pronuclear stage. Enlarged images (X3) of the control and Tle6 Null zygotes indicated the thickness of cortical F-actin. The red bar showed the thickness of cortical F-actin. Scale bar, 20 μm. ( d ) Bar graph (mean±s.e.m.) of cortical F-actin thickness at mitotic zygotes from control and Tle6 Null females. Embryo number was 25 (control) or 20 ( Tle6 Null ). *** P <0.001 indicates statistically significant differences using Student’s t -test. ( e ) Mouse zygotes from control and Tle6 Null females were recovered as in a and stained with DNase I labelled with Alexa Fluor 488 (G-actin, green), phalloidin labelled with Alexa Fluor 546 (F-actin, red) and rabbit anti-TLE6 antibody (TLE6, magenta). G-actin was used as a Rainbow Indicator to depict the intensity of fluorescence. Scale bar, 20 μm. Full size image The SCMC regulates F-actin via Cofilin in mouse zygotes The actin cytoskeleton is a dynamic structure regulated at multiple levels by interacting proteins including Cofilin, Profilin, Arp2/3, Fmn2 and CDC42. To investigate how the SCMC regulates F-actin, we stained mouse zygotes from SCMC null females with protein-specific antibodies. The expression pattern of Arp2, Fmn2 and CDC42 in the subcortex of Tle6 Null zygotes was similar to that in controls ( Supplementary Fig. 6a–c ). However, Cofilin was less concentrated in the subcortex and more diffusely present in the cytoplasm of zygotes from Tle6 Null females compared with normal controls ( Supplementary Fig. 6d ). The changed localization of Cofilin was also observed in zygotes from Floped Null females ( Supplementary Fig. 6d ). On immunoblots, Cofilin, Profilin, Arp2, Arp3 and CDC42 were detected at similar levels in the oocytes and zygotes from SCMC null mice compared with controls ( Fig. 7a ; Supplementary Fig. 6e,f ). Phosphorylated, but not un-phosphorylated Cofilin, was significantly decreased in SCMC null eggs and zygotes ( Fig. 7a,b ) including those mitotic zygotes from Tle6 Null females ( Fig. 7c and Supplementary Fig. 6g ). 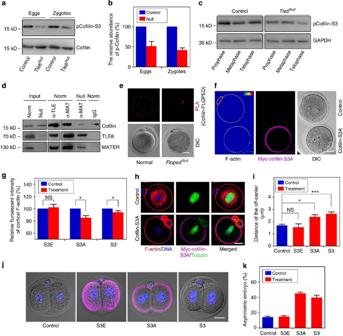Figure 7: The SCMC regulates F-actin through Cofilin. (a) Immunoblots of egg and zygote lysates at similar stages from control andTle6Nullfemale with Cofilin and pCofilin antibody. (b) Relative abundance (mean±s.e.m.) of pCofilin in control and SCMCNulleggs and zygotes was determined by intensity of immunoblot from four independent experiments. Controls were set as 100%. (c) Western blot of pCofilin during mitotic zygotes (synchronous) from control andTle6Nullfemales. (d) Co-IP of Normal (Norm) andMaterNullegg lysates with TLE6 (α-TLE) or MATER (α-MAT) antibodies. Input, egg lysates from normal andMaterNullfemales; IgG, normal rabbit IgG; Norm, normal egg lysates. (e)In situCofilin–FLOPED interactions were detected by PLA using their antibodies.FlopedNullZygote (negative control); Scale bar, 20 μm. (f) Normal interphase zygotes were injected with buffer or mRNA of Myc-confilin-S3A (S3A), and cultured for 4–7 h. After fixation, embryos were mixed and stained with Myc antibody and phalloidin. Myc staining was used to distinguish zygotes from control (buffer) or embryos injected with S3A. Scale bar, 20 μm. (g) Relative immunofluorescent intensity (mean±s.e.m.) of subcortical F-actin in paired zygotes from control and zygotes expressing S3A, Myc-Cofilin-S3E (S3E) or treated with S3 peptides (S3). S3-treated embryo was distinguished from control by pre-staining with TLE6 antibody. Number of paired embryos for S3A, S3E and S3 was 17 (two experiments), 27 (two experiments) and 31 (six experiments), respectively. *P<0.05 indicates statistically significant differences using Student’st-test; NS, no statistically significant differences. (h) Zygotes were treated as inf, but cultured to metaphase and stained. Scale bar, 20 μm. (i) Zygotes were treated as ingand cultured to metaphase. Spindle position (mean±s.e.m.) was calculated as inFig. 4c. Embryo numbers were 33 (S3A, six experiments), 10 (S3E, two experiments) and 61 (S3, nine experiments). *P<0.05; ***P<0.001 indicates statistically significant differences using Student’st-test. (j) Zygotes were treated as ing, and cultured to develop into two-cell embryos and stained. Scale bar, 20 μm. (k) Percent (mean±s.e.m.) of two-cell embryos with asymmetric division was calculated as inFig. 4aafter the treatment as ing(three independent samples). Figure 7: The SCMC regulates F-actin through Cofilin. ( a ) Immunoblots of egg and zygote lysates at similar stages from control and Tle6 Null female with Cofilin and pCofilin antibody. ( b ) Relative abundance (mean±s.e.m.) of pCofilin in control and SCMC Null eggs and zygotes was determined by intensity of immunoblot from four independent experiments. Controls were set as 100%. ( c ) Western blot of pCofilin during mitotic zygotes (synchronous) from control and Tle6 Null females. ( d ) Co-IP of Normal (Norm) and Mater Null egg lysates with TLE6 (α-TLE) or MATER (α-MAT) antibodies. Input, egg lysates from normal and Mater Null females; IgG, normal rabbit IgG; Norm, normal egg lysates. ( e ) In situ Cofilin–FLOPED interactions were detected by PLA using their antibodies. Floped Null Zygote (negative control); Scale bar, 20 μm. ( f ) Normal interphase zygotes were injected with buffer or mRNA of Myc-confilin-S3A (S3A), and cultured for 4–7 h. After fixation, embryos were mixed and stained with Myc antibody and phalloidin. Myc staining was used to distinguish zygotes from control (buffer) or embryos injected with S3A. Scale bar, 20 μm. ( g ) Relative immunofluorescent intensity (mean±s.e.m.) of subcortical F-actin in paired zygotes from control and zygotes expressing S3A, Myc-Cofilin-S3E (S3E) or treated with S3 peptides (S3). S3-treated embryo was distinguished from control by pre-staining with TLE6 antibody. Number of paired embryos for S3A, S3E and S3 was 17 (two experiments), 27 (two experiments) and 31 (six experiments), respectively. * P <0.05 indicates statistically significant differences using Student’s t -test; NS, no statistically significant differences. ( h ) Zygotes were treated as in f , but cultured to metaphase and stained. Scale bar, 20 μm. ( i ) Zygotes were treated as in g and cultured to metaphase. Spindle position (mean±s.e.m.) was calculated as in Fig. 4c . Embryo numbers were 33 (S3A, six experiments), 10 (S3E, two experiments) and 61 (S3, nine experiments). * P <0.05; *** P <0.001 indicates statistically significant differences using Student’s t -test. ( j ) Zygotes were treated as in g , and cultured to develop into two-cell embryos and stained. Scale bar, 20 μm. ( k ) Percent (mean±s.e.m.) of two-cell embryos with asymmetric division was calculated as in Fig. 4a after the treatment as in g (three independent samples). Full size image Co-localization of the SCMC with Cofilin in the subcortex of mouse zygotes and Cofilin-related defects in SCMC null zygotes prompted investigation of physical interactions between the two. Although Cofilin was weakly co-immunoprecipitated by rabbit anti-TLE6 antibody from ovarian lysates ( Supplementary Fig. 6h ), Cofilin was specifically pulled down by TLE6 and MATER antibodies from the lysate of normal eggs ( Fig. 7d ). This direct interaction was substantiated by a proximal ligation assay using Cofilin and FLOPED antibodies, which primarily located the interaction in the periphery of zygotes from normal, but not Floped Null , female mice ( Fig. 7e ). Taken together, these data suggest that the SCMC regulates subcortical F-actin through Cofilin, a known regulator of actin cytoskeleton [29] . Cofilin is required for the symmetrical division of zygotes Increased Cofilin activity has been shown to cause rapid regression of the cleavage furrow and inhibit further cleavage in Xenopus zygotes [30] . To investigate the role of Cofilin in mouse pre-implantation development, we injected zygotes with a constitutively active mutant of Cofilin (Cofilin-S3A, in which Cofilin at Ser3 was replaced with alanine) and an inactive mutant S3E (Cofilin-S3E, in which Cofilin at Ser3 was replaced with glutamine) [31] , [32] . The immunofluorescent intensity of subcortical F-actin was significantly decreased in zygotes injected with the mRNA of Myc-Cofilin-S3A, but not in zygotes injected with Myc-Cofilin-S3E when paired zygotes were compared ( Fig. 7f,g ). The injection of Cofilin-S3A, but not Cofilin-S3E, disrupted the cytoplasmic F-actin meshwork and the central position of spindle in mouse zygotes ( Fig. 7h,i ), and resulted in asymmetric two-cell embryos ( Fig. 7j,k ). We further treated mouse zygotes with a cell-permeable synthetic peptide (S3 peptide) that contains the phosphorylation site of Cofilin and competitively inhibits phosphorylation of the endogenous protein [33] . The embryos treated with the S3 peptide had defects similar to those injected with Cofilin-S3A ( Fig. 7g,i–k ). Thus, these results indicate that Cofilin plays an important role in the actin cytoskeleton that centrally positions the spindle in mouse zygotes. Only a limited number of maternal effect genes (<30) have been characterized in mammals, which reflects technological limitations, including the paucity of eggs and early embryos, that complicate molecular investigations [6] , [34] . We recently identified a SCMC that is specifically expressed in mammalian oocyte–embryos and minimally includes FLOPED, MATER, Filia and TLE6 proteins [14] . Although FILIA, which contains a KH domain, has been shown to interact with RNAs [35] , the molecular functions of the proteins in SCMC are largely unknown. TLE6 regulates gene expression by interacting with BF-1 as a co-repressor of TLE1 in neural progenitors [20] . However, TLE6 does not localize in the nucleus of mouse oocytes and early embryos. Herein, we have documented that the absence of TLE6 disrupts the SCMC and adversely affects the F-actin cytoskeleton, leading to asymmetric cell division and cleavage-stage embryonic death. The actin cytoskeleton forms different structures depending on interacting proteins and at least 15 distinct F-actin structures have been documented in metazoan cells [36] . Because eggs and early embryos are unique [37] , the presence of specific components for regulating their actin cytoskeletons is anticipated in these cells. Earlier studies, using F-actin affinity chromatography, identified novel F-actin-binding proteins in eggs and embryos of Drosophila melanogaster and Caenorhabditis elegans [38] , [39] . The functional characterization of these proteins has provided insights into the role of F-actin cytoskeleton [40] , [41] . Cofilin plays a central role in modulating F-actin dynamics and is commonly present in highly dynamic F-actin structures observed in locomotory and invasive protrusions of motile cells [29] , [42] . Cofilin has been also shown to increase the concentration of G-actin by promoting F-actin depolymerization, which contributes to F-actin assembly [43] . Whether Cofilin promotes polymerization or depolymerization depends on its concentration relative to actin and the presence of other actin-binding proteins [29] . In normal mouse zygotes, Cofilin is primarily located in the subcortex [44] and we now document that it interacts and co-localizes with the SCMC. The absence of the SCMC affects the activity and the localization of Cofilin, but not other F-actin regulators. The decreased subcortical F-actin, increased G-actin and thickened cytoplasmic F-actin bundles suggests that increased activity of Cofilin disrupts actin filaments, which leads to the off-centre spindle observed in the SCMC null mutants. Recently, Xenopus ADF/Cofilin and its activator, Slingshot phosphatase, have been identified as key regulators of actin dynamics essential for spindle microtubule assembly during Xenopus oocyte maturation [45] . Thus, the SCMC may regulate spindle assembly by controlling F-actin dynamics through Cofilin in mouse zygotes. The cytoplasmic F-actin network was previously observed in Drosophila syncytial embryos [46] and in starfish oocytes where, during meiosis, M-phase microtubules are short relative to the 180-μm-diameter oocyte [47] . Subsequently, several groups reported that cytoplasmic F-actin networks play critical roles in the meiosis of mouse oocytes [48] , [49] , [50] . Although the absence of cytoplasm F-actin network results in the defect of spindle translocation in Mater Null (ref. 51 ), oocytes from these mice undergo normal meiosis and the ovulated eggs can be fertilized, implying that the SCMC and the cytoplasm F-actin network play relatively modest roles in the maturation of mouse oocytes. A specific Arp2/3-dependent F-actin domain in the cortex of mouse oocytes was reported to be required for asymmetrical spindle position during meiosis [28] . However, subcortical F-actin and Arp2/3 proteins were not affected in oocytes from SCMC mutant female mice. These observations suggest that different pathways may be required to coordinately regulate spindle location during mouse oogenesis and early embryonic development. Although the SCMC interacts with F-actin and Cofilin, we have not yet detected direct in vitro binding of Cofilin with any individual component of the SCMC. However, the molecular mass of the SCMC is between ~669 and 2,000 kDa, which is much larger than the aggregate mass (~250 kDa) of the known proteins [34] . Thus, the presence of additional proteins in the SCMC is likely and one or more of them could directly interact with Cofilin in the regulating F-actin polymerization. Taken together, our results demonstrate that Tle6 is a novel maternal effect gene that is essential for mouse early embryonic development. A primary role of the TLE6 protein is to stabilize the SCMC that controls Cofilin regulation of F-actin dynamics to ensure symmetric cell division and proper cell division of mouse zygotes. Similar mechanisms may play important roles in human early embryonic development, defects of which will result in the arrest of embryonic development and human infertility. Mouse lines and establishment of transgenic mice SCMC mutant mouse lines were maintained in compliance with the guidelines of the Animal Care and Use Committee of the Institute of Zoology at the Chinese Academy of Sciences (CAS). To generate Tle6 mutant mice, the targeting vector contained a neomycin-resistant cassette that replaced the transcription and translational start sites, as well as the first two exons of the coding region of Tle6 was constructed using DNA recombineering ( Supplementary Fig. 1d ). Successfully targeted heterozygous ES cells were identified by PCR with specific primers and confirmed by Southern hybridization of Nhel -digested genomic DNA using probes immediately 5′ and 3′ to the targeting vector ( Supplementary Fig. 1e,f ). Two clones (#107 and #111) from successfully targeted heterozygous ES cell lines were injected into blastocyst embryos to establish transgenic mouse lines. Two male chimera were used for germ line transmission of the targeted allele ( − ) and subsequent genotyping was determined by PCR products of mouse genomic DNA. P1 (5′- actctaacccaggccatcct -3′) and P2 (5′- tcagcaggtgaaggtgattg -3′) were used to detect the normal (+) allele (875 bp), and primers P1 and P3 (5′- cagaaagcgaaggagcaaag -3′) were used to detect the null (−) allele (449 bp) in PCR genotyping. Conditions for the PCR were: 1 cycle at 94 °C for 4 min; 40 cycles at 94 °C for 30 s, 60 °C for 30 s and 72 °C for 1 min, and a final extension at 72 °C for 10 min. Genomic DNA from the tail of +/+, +/− and −/− mice was sequenced to confirm proper homologous recombination. The successful depletion of Tle6 was further confirmed by the absence of mRNA (reverse transcription PCR (RT–PCR)) and proteins in the ovaries and oocytes from Tle6 −/− female mice ( Fig. 2a–c ). Collection of eggs and embryos and assessment of fertility Female mice (6–8 week old) were stimulated with gonadotrophins to obtain ovulated eggs or embryos at defined times. Ovulated eggs and embryos were collected in M2 medium and either imaged or snap frozen for storage at −80 °C prior to biochemical analyses. Timed embryos were collected in M2 medium and cultured in KSOM (Merck Millipore) at 37 °C in 5% CO 2 . Zygotes were treated with the S3 fragment peptide that contains the phosphorylation site of Cofilin and competitively inhibits phosphorylation of endogenous ADF/Cofilin (AnaSpec, Fremont, CA, USA; 5 mg ml −1 in DMSO as the stock solution). Periodic acid-Schiff’s staining was performed as previously described [14] . Briefly, ovaries from heterozygous and homozygous Tle6 mice were fixed, embedded in polymethyl methacrylate, sectioned and stained with periodic acid-Schiff’s reagents. Commercially obtained ICR and C57BL/6J mice were used as normal controls. In vivo fertility was assessed by 2:1 caging of one Tle6 +/− (control) and one Tle6 Null female with individual Tle6 +/+ , Tle6 +/− or Tle6 Null male for over 3 months. Successful matings were verified by the presence of a post-coital vaginal plug after which females were caged separately. More than five independent cages were set for the experiment. Immunoblots and immunohistochemistry Primary antibodies included: rabbit anti-FLOPED (1:1,000 for western blot, 1:500 for immunohistochemistry), rabbit anti-TLE6 (1:1,000 for western blot, 1:500 for immunohistochemistry), rabbit anti-MATER (1:5,000 for western blot, 1:1,000 for immunohistochemistry) and sheep anti-FILIA (1:1,000 for western blot, 1:200 for immunohistochemistry ) [14] , mouse monoclonal antibody to MATER (1:500) generated by Abmart (Shanghai, China), mouse monoclonal anti-GAPDH (1:3,000, Abmart), mouse monoclonal antibody to α-tubulin (1:200, FITC-conjugated, Sigma-Aldrich), rabbit anti-CDC42 (1:1,000), rabbit anti-Cofilin-1 (1:1,000 for western blot, 1:100 for immunohistochemistry), rabbit anti-phospho-Cofilin 1 (Ser3, 1:1,000), rabbit anti-myc (1:200) and rabbit anti-Profilin 1 (1:1,000; Cell Signalling Technology, Danvers, MA, USA), mouse monoclonal anti-pan-actin (1:200), rabbit anti-Arp2 (1:1,000 for western blot, 1:200 for immunohistochemistry), mouse monoclonal anti-Arp3 (1:1,000) and rabbit anti-Fmn2 (1:200) (Abcam, Cambridge, MA, USA) and rabbit anti-CDC42 (1:50, Santa Cruz, for immunofluorescence). The secondary antibodies included: goat anti-mouse conjugated with Alexa Fluor 488 (1:200), donkey anti-rabbit conjugated with Alexa Fluor 488 (1:1,000), donkey anti-rabbit conjugated with Alexa Fluor 633 (1:1,000), donkey anti-sheep conjugated with Alexa Fluor 488 (1:500) (Invitrogen, Life Technologies, Grand Island, NY, USA), donkey anti-rabbit, -sheep conjugated with horseradish peroxidase (HRP) (1:1,000, Jackson ImmunoResearch, West Grove, PA, USA) and goat anti-mouse with HRP (1:1,000, Abmart). Samples for immunoblots were prepared with SDS sample buffer, separated by NuPAGE 4–12% SDS–PAGE and transferred to PVDF membranes (Invitrogen). The blots were pre-treated with Superblock Blocking Buffer (Pierce, Thermo Fisher Scientific, Rockford, IL, USA), incubated (4 °C, overnight) with primary antibodies, washed once with PBST [14] and incubated (1 h, room temperature (RT)) with HRP-conjugated secondary antibodies. Immunoreactivity was detected with SuperSignal West Dura Extended Duration Substrate (Pierce). Images of the blots were obtained by using a Bio-RAD Chemi DocTMXR s+ (Bio-Rad Laboratories,USA) with Image Lab software. Immunohistochemistry was performed with EnVision G/2 System/AP (DAKO, Carpinteria, CA, USA) according to the manufacturer’s protocol. Immunofluorescent staining for mouse eggs and embryos was modified from a previously reported protocol [52] . In brief, eggs and embryos were fixed with 130 mM KCl, 25 mM HEPES (pH 7.0), 3 mM MgCl 2 , 4% paraformaldehyde, 0.15% glutaraldehyde, 0.06% Triton X-100, permeabilized in PBS containing 0.5% Triton X-100, blocked with 5% donkey serum and 0.1% BSA in PBS at RT for 1 h, incubated (over night, 4 °C) with primary antibodies followed by secondary antibody (1 h, RT). F-actin, G-actin and DNA were detected with Alexa Fluor 546-labelled phalloidin, DNase I labelled with Alexa Fluor 488 and Hoechest (Invitrogen), respectively. Alternatively, eggs and embryos were recovered together with oviducts, processed as above and sectioned (4 μm) prior to immunostaining. Immunofluorescent images were obtained on an Axioplan Zeiss microscope (LSM 780, Carl Zeiss, Thornwood, NY, USA) and the intensity of immunofluorescent signal was analyzed with ZEN lite 2011 (Carl Zeiss). Protein–protein interactions Co-immunoprecipitation (Co-IP) of ovarian lysate was performed with ProFoundTM Mammalian Co-Immunoprecipitation Kit (Pierce) according to the manufacturer’s protocol. Briefly, antibody coupling gel was conjugated with specific antibodies, incubated (1–1.5 h, RT) with ovarian lysates, washed with PBST and eluted with elution buffer. Co-IP products were further analyzed by immunoblot. Precleared egg lysate from normal and Tle6 or mater null eggs (150) was precipitated as described previously with protein G-Separose beads (Santa Cruz, G2613) by using TLE6 and MATER antibodies [16] . Mouse immunoglobulin G was used as the negative control. In situ detection of protein–protein interaction was performed by PLA according to the manufacturer’s protocol using the DuolinkII Detection Kit with PLA PLUS and MINUS Probes for rabbit antibodies (Olink Bioscience, Sigma-Aldrich). Rabbit anti-FLOPED, anti-TLE6, anti-Cofilin-1 antibodies were conjugated with PLA PLUS, PLA MINUS and PLA MINUS probes, respectively. The zygotes from Floped Null and Tle6 Null females were used as negative controls. Plasmid construction, microinjection and time-lapse imaging The vectors pCS2-Myc-confilin S3E and Cofilin-S3A were amplified from mouse ovarian complementary DNA (cDNA) with the primers (Cofilin-S3E forward primer, 5′- ttcaggccggccgatggccGAAggtgtggctgt -3′; Cofilin-S3A forward primer, 5′- ttcaggccggccgatggccGCTggtgtggctgt -3′; reverse primer, 5′- ttaaggcgcgcctcacaaaggcttgccct -3′). The pCS2-Tle6–eGFP was cloned from mouse ovarian cDNA with the primers ( Tle6 forward primer, 5′- ttccccgcggatgacttcccacagacagag -3′; Tle6 reverse primer, 5′- cgggaccggtaacaggtacttgatgtggta -3′). The pUtrCH–eGFP and pRN3-β5-tubulin–GFP were from Addgene ( http://www.addgene.org/ ) and Dr Marie-Hélène Verlhac, respectively. The transcripts (mRNA) of Myc-Cofilin-SA, Myc-Cofilin-S3E, β5-tubulin–GFP [26] , UtrCH–eGFP [27] and Tle6–eGFP were prepared in vitro using linearized plasmid with a mMessage mMachine kit (Ambion). About 5–10 pl of the β -5-tubulin–GFP , UtrCH–eGFP and Tle6–eGFP mRNA purified with the RNeasy MinElute Cleanup Kit (Qiagen, Valencia, CA, USA) were microinjected into the cytoplasm of zygotes and cultured in KSOM at 37 °C in 5% CO 2 for 4–8 h. Hoechst 33342 (Invitrogen) was used to stain DNA. After developing into the appropriate stages, the injected zygotes were recovered for further experiments (time-lapse imaging or immunostaining). The time-lapse images of β5-Tubulin–GFP, UtrCH–eGFP and TLE6–eGFP were processed by the Velocity software 6.0.1 (Perkin Elmer) after the zygotes were imaged with the UltraVIEW VoX confocal imaging system (Perkin Elmer). Measurements of cortical F-actin were modified from a previous report [28] . Briefly, the confocal images of UtrCH–eGFP were obtained at 37 °C in 5% CO 2 , KSOM medium, using a Plan APO 60X/1.4 UC PFS OIL objective with a Nikon microscope. One focal plane corresponding to the embryo's largest diameter in the unsaturated images was measured with the Velocity software 6.0.1 (Perkin Elmer). Each embryo was measured four times and the mean value was reported as the thickness of cortical F-actin. RNA quantitation and expression Total RNA was isolated from Tle6 +/− and Tle6 Null mouse ovaries using an RNeasy Mini Kit (Qiagen). Contaminating genomic DNA was removed by digestion with RNase-free DNase I (Qiagen) and RNA was reverse transcribed to cDNA using the Superscript III First Strand System (Invitrogen). The OneStep RT–PCR Kit (Qiagen) was used in semi-quantitative RT–PCR to assess the abundance of normal and mutant Tle6 transcripts in Tle6 mutant mice (forward primer: 5′- ggtggacttaatcagatttgtgacc -3′ and reverse primer: 5′- aattgccagagtgctgtgcta -3′). Gapdh was amplified as a control of RNA integrity (forward primer: 5′- accacagtccatgccatcac -3′ and reverse primer: 5′- tccaccaccctgttgctgta -3′). Quantitative real-time RT–PCR was used to determine the abundance of Tle6, Floped, Filia and Mater transcripts using TaqMan probes and gene-specific primers (Mm00509585_gl, Mm00475107_m1 and Mm00488691_ml) and GAPDH (Applied Biosystems, Foster City, CA, USA) as an endogenous control for normalization. Each data point was the average of duplicate assays performed on three independently obtained biological samples and expressed as a per cent of Gapdh abundance (mean±s.e.m.). Statistical analyses Quantitative analyses were based on at least 3–5 independent biological samples and expressed as the mean±s.e.m. Statistical analyses were carried out using Student’s t -test for comparing the difference between two groups that showed normal (Gaussian) distribution with GraphPad Prism software, with P -values <0.05 considered significant. How to cite this article: Yu, X.-J. et al . The subcortical maternal complex controls symmetric division of mouse zygotes by regulating F-actin dynamics. Nat. Commun. 5:4887 doi: 10.1038/ncomms5887 (2014).